Substrate ectodomain is critical for substrate preference and inhibition of γ-secretase Understanding the substrate recognition mechanism of γ-secretase is a key step for establishing substrate-specific inhibition of amyloid β-protein (Aβ) production. However, it is widely believed that γ-secretase is a promiscuous protease and that its substrate-specific inhibition is elusive. Here we show that γ-secretase distinguishes the ectodomain length of substrates and preferentially captures and cleaves substrates containing a short ectodomain. We also show that a subset of peptides containing the CDCYCxxxxCxCxSC motif binds to the amino terminus of C99 and inhibits Aβ production in a substrate-specific manner. Interestingly, these peptides suppress β-secretase-dependent cleavage of APP, but not that of sialyltransferase 1. Most importantly, intraperitoneal administration of peptides into mice results in a significant reduction in cerebral Aβ levels. This report provides direct evidence of the substrate preference of γ-secretase and its mechanism. Our results demonstrate that the ectodomain of C99 is a potent target for substrate-specific anti-Aβ therapeutics to combat Alzheimer’s disease. The γ-secretase complex, which comprises four membrane proteins, hydrolyses the transmembrane domain of type I membrane proteins in the hydrophobic environment of the lipid bilayer [1] , [2] , [3] , [4] , [5] , [6] , [7] , [8] . β-Amyloid precursor protein (APP) is the best-studied substrate of this protease, as its carboxyl terminal fragment (referred to as C99) is generated by β-secretase. C99 is a direct substrate of γ-secretase and is processed into amyloid β-protein (Aβ), a known culprit in the pathogenesis of Alzheimer’s disease (AD) [9] , [10] , [11] . Inhibition of γ-secretase is among the most effective approaches for suppressing Aβ production. However, its inhibition can cause cleavage defects of numerous membrane proteins including Notch [12] , [13] . On the other hand, γ-secretase modulators (GSMs) are promising drugs for decreasing Aβ42 production without affecting Notch processing [14] , [15] ; however, it was recently reported that GSM-1 showed limited efficacy on γ-secretase in patients with mild cognitive impairment/AD [16] . Thus, the development of substrate-specific inhibition of γ-secretase is highly desirable. β-Secretase is also a promising drug target for anti-amyloid therapeutics for reducing C99 production [17] , [18] . However, as in the case of γ-secretase, β-secretase hydrolyses a number of membrane proteins, such as close homologue of L1, contactin-2, L1, neuregulin-1, seizure-protein 6, sialyltransferase 1 (St6gal1), vascular endothelial growth factor receptor 1 and voltage-gated sodium channels [19] , [20] , [21] , [22] , [23] , [24] , [25] . β-Secretase-deficient mice exhibited hypomyelination of peripheral nerves, delayed remyelination, axonal bundling abnormalities, schizophrenic symptoms, retinal thinning, reduction of retinal vascular density, increase of lipofuscin and sodium channel activation [20] , [21] , [26] , [27] , [28] , [29] , [30] . These indicate that pharmacological inhibition of β-secretase should be performed in a substrate-specific manner. In this study, we directly demonstrate that γ-secretase distinguishes the ectodomain length of substrates and preferentially captures and cleaves substrates containing a short ectodomain. Based on the substrate recognition mechanism of γ-secretase, we propose that blocking the C99 ectodomain is a potent approach for substrate-specific dual inhibition of β- and γ-secretases. C99 is an inefficient substrate for γ-secretase Understanding the substrate recognition mechanism of γ-secretase is a key step to establishing substrate-specific inhibition of Aβ production. In order to investigate the substrate recognition mechanism of this protease, first we examined the substrate selectivity of γ-secretase. We generated recombinant γ-secretase substrates containing the native N-terminus sequence by using the Profinity eXact protein purification system [31] ( Fig. 1 ). A CHAPSO-solubilized microsomal fraction from HEK cells was incubated with C99-FLAG and C83-FLAG substrates, and productions of APP intracellular domain (AICD) were analysed with defined amounts of FLAG-tagged AICD (AICD–FLAG) by western blotting [32] . We found that AICD production from C83-FLAG was much greater than that from C99-FLAG, suggesting that C99 is an inefficient substrate for proteolysis by γ-secretase ( Fig. 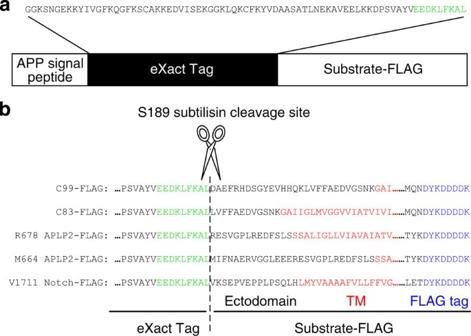Figure 1: Schematic diagrams of generating γ-secretase substrates. γ-Secretase substrates were expressed as fusion proteins with the APP signal peptide and the Profinity eXact tag (Bio-Rad) in sf9 cells (a). The Profinity eXact tag protein purification system offers purification of recombinant proteins with a native amino terminus. Once Profinity eXact-tagged γ-secretase substrates were captured using S189 subtilisin-immobilized resin, addition of sodium fluoride triggered precise cleavage at the carboxyl terminus of the cleavage-recognition sequence (shown in green) and the release of substrates with abona fideN terminus. Purified substrates were recaptured using anti-FLAG M2 agarose beads (Sigma) and eluted by addition of 0.2 M glycine, pH 2.7 and 0.3% NP40. 1/10th volume of 3 M Tris-HCl, pH 8.0 was added to the eluted substrates for neutralization. The flanking region of the S189 subtilisin cleavage site in each substrate is shown inb. 2a and Table 1 ; Supplementary Fig. S14 ). The difference between C99-FLAG and C83-FLAG lies, in principle, in the ectodomain length. To test whether substrate length and extension of its C-terminus influence the cleavage efficiency of γ-secretase, we generated the C83 substrate extended by 16 residues at its C terminus (C83-GS-FLAG, 99 amino acids) ( Fig. 3a,b ; Supplementary Fig. S15 ). C83-GS-FLAG exhibited an indistinguishable cleavage rate from the original C83-FLAG. These data suggest that total substrate length and C-terminal length are not critical for cleavage efficiency of γ-secretase. We also observed that levels of Aβ and AICD produced from C99 substrates containing tandem repeats of FLAG tags at its C terminus (C99-3X FLAG and C99-5X FLAG) were indistinguishable from those of original C99-FLAG ( Fig. 3c,d ; Supplementary Fig. S15 ). These data suggest that total substrate length and C-terminus length are not critical for ε-cleavage efficiency and that the ectodomain length of the substrate influences the cleavage efficiency of γ-secretase. Figure 1: Schematic diagrams of generating γ-secretase substrates. γ-Secretase substrates were expressed as fusion proteins with the APP signal peptide and the Profinity eXact tag (Bio-Rad) in sf9 cells ( a ). The Profinity eXact tag protein purification system offers purification of recombinant proteins with a native amino terminus. Once Profinity eXact-tagged γ-secretase substrates were captured using S189 subtilisin-immobilized resin, addition of sodium fluoride triggered precise cleavage at the carboxyl terminus of the cleavage-recognition sequence (shown in green) and the release of substrates with a bona fide N terminus. Purified substrates were recaptured using anti-FLAG M2 agarose beads (Sigma) and eluted by addition of 0.2 M glycine, pH 2.7 and 0.3% NP40. 1/10th volume of 3 M Tris-HCl, pH 8.0 was added to the eluted substrates for neutralization. The flanking region of the S189 subtilisin cleavage site in each substrate is shown in b . 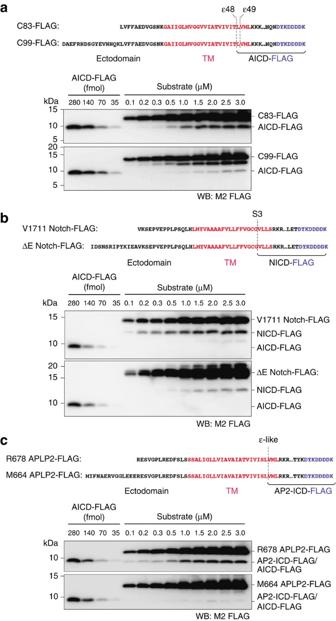Figure 2: Substrate preference of γ-secretase. C83-FLAG and C99-FLAG substrates were incubated with a CHAPSO-solubilized CHO microsomal fraction to evaluate the substrate preference of γ-secretase (a). C83-FLAG was efficiently cleaved to produce AICD–FLAG compared with inefficient cleavage of C99-FLAG. Dashed lines indicate ε-cleavage sites. V1711 Notch-FLAG containing a native N terminus is a shorter substrate and was efficiently cleaved to produce NICD–FLAG compared with inefficient cleavage of ΔE Notch-FLAG (b). The dashed line indicates the S3 cleavage site. M664 APLP2-FLAG and R678 APLP2-FLAG are analogous to β- and α-cleaved substrates, respectively (c). R678 APLP2-FLAG possesses a short ectodomain and was efficiently cleaved by γ-secretase to produce AP2-ICD-FLAG compared with inefficient cleavage of M664 APLP2-FLAG. Dashed lines indicate cleavage sites. Full size image Figure 2: Substrate preference of γ-secretase. C83-FLAG and C99-FLAG substrates were incubated with a CHAPSO-solubilized CHO microsomal fraction to evaluate the substrate preference of γ-secretase ( a ). C83-FLAG was efficiently cleaved to produce AICD–FLAG compared with inefficient cleavage of C99-FLAG. Dashed lines indicate ε-cleavage sites. V1711 Notch-FLAG containing a native N terminus is a shorter substrate and was efficiently cleaved to produce NICD–FLAG compared with inefficient cleavage of ΔE Notch-FLAG ( b ). The dashed line indicates the S3 cleavage site. M664 APLP2-FLAG and R678 APLP2-FLAG are analogous to β- and α-cleaved substrates, respectively ( c ). R678 APLP2-FLAG possesses a short ectodomain and was efficiently cleaved by γ-secretase to produce AP2-ICD-FLAG compared with inefficient cleavage of M664 APLP2-FLAG. Dashed lines indicate cleavage sites. Full size image Table 1 Apparent K m and V max values for each substrate. 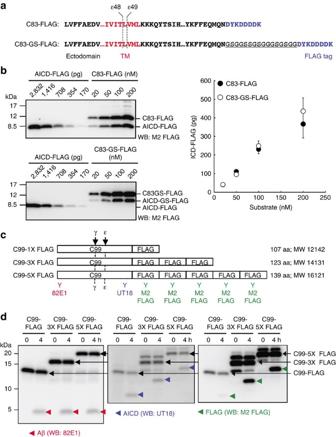Figure 3: Length of substrate C terminus is not critical for the cleavage efficiency. A GS-stretch (of 16-residues) was inserted prior to the FLAG tag to generate C83-GS-FLAG, a 99-residue substrate tagged FLAG sequence (equivalent in length to C99-FLAG) (a). C83-GS-FLAG was incubated with γ-secretase fraction and subjected to western blotting to visualize AICD–FLAG production (b). C83-GS-FLAG exhibited an indistinctive cleavage compared with C83-FLAG cleavage. Tandem repeats of FLAG tag were inserted at C99 C terminus to examine the effect of extension of intracellular domain length on cleavage efficiency (c). Attachment of tandem repeats of FLAG tags failed to alter production of Aβ and AICD (d). Full size table Figure 3: Length of substrate C terminus is not critical for the cleavage efficiency. A GS-stretch (of 16-residues) was inserted prior to the FLAG tag to generate C83-GS-FLAG, a 99-residue substrate tagged FLAG sequence (equivalent in length to C99-FLAG) ( a ). C83-GS-FLAG was incubated with γ-secretase fraction and subjected to western blotting to visualize AICD–FLAG production ( b ). C83-GS-FLAG exhibited an indistinctive cleavage compared with C83-FLAG cleavage. Tandem repeats of FLAG tag were inserted at C99 C terminus to examine the effect of extension of intracellular domain length on cleavage efficiency ( c ). Attachment of tandem repeats of FLAG tags failed to alter production of Aβ and AICD ( d ). Full size image Substrate preference of γ-secretase To confirm the effect of substrate ectodomain length on γ-secretase-dependent cleavage, we generated Notch and APP-like protein 2 (APLP2) substrates containing different ectodomain lengths and examined their cleavage efficiency ( Fig. 2b,c ). As observed for C99-FLAG, Notch substrate containing an extended N-terminal sequence (ΔE Notch-FLAG) was an inefficient substrate with which to produce a Notch intracellular domain (NICD) compared with V1711 Notch-FLAG containing a bona fide S2 cleaved ectodomain sequence ( Fig. 2b and Table 1 ; Supplementary Fig. S14 ) [33] , [34] , [35] . The APLP2 substrate containing a long ectodomain (M664 APLP2-FLAG; β-cleaved) exhibited a less efficient cleavage for producing an APLP2 intracellular domain (AP2-ICD) compared with a substrate having a short ectodomain (R678 APLP2-FLAG; α-cleaved) ( Fig. 2c and Table 1 ; Supplementary Fig. S14 ) [36] . It is important to note that V max / K m values of substrates containing short ectodomains (C83-FLAG, V1711 Notch-FLAG and R678 APLP2-FLAG) are roughly fivefold greater than those of long ectodomain substrates (C99-FLAG, ΔE Notch-FLAG and M664 APLP2-FLAG) ( Table 1 ). To confirm the substrate preference of γ-secretase in different reaction conditions, we also examined cleavages of C99-FLAG and V1711 Notch substrates at different time points ( Supplementary Figs S1 and S21 ) and at different concentrations of γ-secretase ( Supplementary Figs S2 and S21 ). In either case, γ-secretase preferentially cleaved V1711 Notch-FLAG. These data indicate that γ-secretase preferentially cleaves substrates containing short ectodomains in general. It is important to note that the ectodomain length does not affect the cleavage sites close to the membrane/cytoplasmic boundary (ε-, S3 and ε-like sites) on the substrates ( Supplementary Fig. S3 ). γ-Secretase distinguishes the substrate ectodomain length To ascertain whether γ-secretase distinguishes the ectodomain of a substrate, we performed ectodomain-swapping experiments using C99 and V1711 Notch substrates ( Fig. 4a ). The ectodomain of C99-FLAG was exchanged with that of V1711 Notch-FLAG and the resultant substrate (V1711 Notch-C99-FLAG) was efficiently cleaved by γ-secretase ( Fig. 4b ; Supplementary Fig. S16 ). Co-immunoprecipitation of the substrate with an M2 FLAG antibody in a CHAPSO-solubilized microsomal fraction revealed that V1711 Notch-C99-FLAG had an increased interaction with γ-secretase components compared with C99-FLAG ( Fig. 4c ; Supplementary Fig. S16 ). By contrast, when Notch-FLAG had its ectodomain exchanged with the C99 ectodomain (C99-Notch-FLAG), NICD production and association with γ-secretase components were significantly decreased compared with V1711 Notch-FLAG ( Fig. 4b,c ; Supplementary Fig. S16 ). These results fit the idea that γ-secretase distinguishes the ectodomain length of substrates by capturing the ectodomain and preferentially cleaves substrates containing a short ectodomain. Indeed, we observed that C83-FLAG interacted with more γ-secretase components, compared with C99-FLAG ( Supplementary Figs S4 and S21 ). Interestingly, we observed non-selective binding of immature nicastrin to substrates used in this assay ( Fig. 4c ; Supplementary Fig. S4 ). However, one may assume that the Aβ1–16 sequence, rather than its length in C99, is inhibitory for recognition and cleavage by γ-secretase. To exclude the possibility that the Aβ1–16 sequence in C99 possesses inhibitory effects on cleavage and recognition by γ-secretase, we generated a C99-FLAG substrate containing a reverse sequence of Aβ1–16 at the N terminus (RVC99-FLAG) and examined its cleavage and interaction with this enzyme ( Fig. 5a ). RVC99-FLAG exhibited indistinguishable AICD production and interaction with γ-secretase from the original C99-FLAG ( Fig. 5b,c ; Supplementary Fig. S17 ). 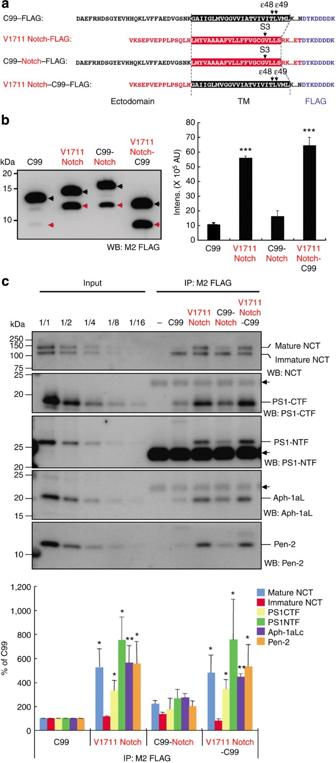Figure 4: Ectodomain swapping of C99 and V1711 Notch substrates. Diagram showing C99, V1711 Notch and their chimeric substrates (a). Black and red indicate C99 and V1711 Notch-derived sequences, respectively. The boxed sequence indicates the transmembrane region of the substrate. Arrows indicate cleavage sites on each substrate. Chimeric substrates were incubated with CHAPSO-solubilized γ-secretase fractions and western blotting was used to visualize and quantify the intracellular domain released from the substrate (b). Substrates containing the ectodomain of V1711 Notch were efficiently cleaved by γ-secretase. Black arrowhead, substrate; red arrowhead, intracellular domain. Intensity of each band of intracellular domain was quantified using LAS-4000 luminescent image analyser and plotted in arbitrary unit. Data are expressed as means±s.d. of three independent experiments. ***P<0.0005 (analysis of variance (ANOVA), Scheffe’spost hoctest compared with C99). Substrates were immobilized using anti-FLAG M2 magnetic beads and mixed with CHAPSO-solubilized γ-secretase fractions (c). After sufficient washing of co-immunoprecipitates, western blotting was used to visualize and quantify γ-secretase components. Substrates containing the ectodomain of V1711 Notch (V1711 Notch-FLAG and V1711 Notch-C99-FLAG) had increased interaction with γ-secretase components. By contrast, substrates containing C99 ectodomain decreased interaction with γ-secretase components. Interestingly, immature nicastrin bound to any substrate equally. Arrows indicate the position of immunoglobulin G used for co-immunoprecipitation. Data are expressed as means±s.d. of three independent experiments. *P<0.05, **P<0.005 (ANOVA, Scheffe’spost hoctest compared with C99). Figure 4: Ectodomain swapping of C99 and V1711 Notch substrates. Diagram showing C99, V1711 Notch and their chimeric substrates ( a ). Black and red indicate C99 and V1711 Notch-derived sequences, respectively. The boxed sequence indicates the transmembrane region of the substrate. Arrows indicate cleavage sites on each substrate. Chimeric substrates were incubated with CHAPSO-solubilized γ-secretase fractions and western blotting was used to visualize and quantify the intracellular domain released from the substrate ( b ). Substrates containing the ectodomain of V1711 Notch were efficiently cleaved by γ-secretase. Black arrowhead, substrate; red arrowhead, intracellular domain. Intensity of each band of intracellular domain was quantified using LAS-4000 luminescent image analyser and plotted in arbitrary unit. Data are expressed as means±s.d. of three independent experiments. *** P <0.0005 (analysis of variance (ANOVA), Scheffe’s post hoc test compared with C99). Substrates were immobilized using anti-FLAG M2 magnetic beads and mixed with CHAPSO-solubilized γ-secretase fractions ( c ). After sufficient washing of co-immunoprecipitates, western blotting was used to visualize and quantify γ-secretase components. Substrates containing the ectodomain of V1711 Notch (V1711 Notch-FLAG and V1711 Notch-C99-FLAG) had increased interaction with γ-secretase components. By contrast, substrates containing C99 ectodomain decreased interaction with γ-secretase components. Interestingly, immature nicastrin bound to any substrate equally. Arrows indicate the position of immunoglobulin G used for co-immunoprecipitation. Data are expressed as means±s.d. of three independent experiments. * P <0.05, ** P <0.005 (ANOVA, Scheffe’s post hoc test compared with C99). 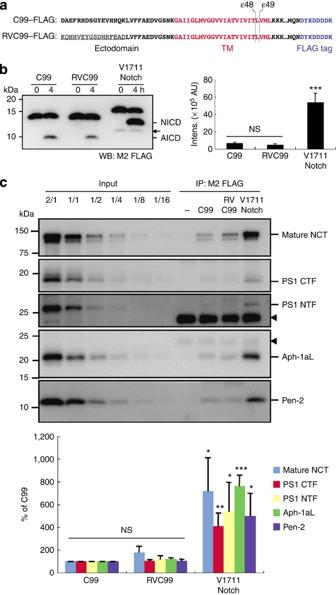Figure 5: Reverse sequence of Aβ1–16 in C99-FLAG exhibited indistinctive cleavage compared with the original C99 substrate. The 1–16 region of C99 was inverted in C99-FLAG substrate (RVC99-FLAG) and we compared its cleavage efficiency with original C99-FLAG (a). Underline, inverted sequence of Aβ1–16. C99, RVC99 and Notch substrates were incubated with a γ-secretase fraction at 37 °C for 4 h. ICD-FLAG fragments were separated on a gel, followed by western blotting with anti-FLAG M2 antibody (b). C99-FLAG substrate containing a reverse sequence of Aβ1–16 in C99 exhibited indistinctive cleavage compared with original C99-FLAG. Arrow indicates a degradation product of the substrate during purification. Data are expressed as means±s.d. of three independent experiments. ***P<0.0005 (analysis of variance, (ANOVA), Scheffe’spost hoctest compared with C99). NS, not significant. Substrates were immobilized using anti-FLAG M2 magnetic beads and mixed with γ-secretase fractions (c). After sufficient washing of co-immunoprecipitates, western blotting was used to visualize and quantify γ-secretase components. RVC99-FLAG showed indistinctive interaction with γ-secretase components compared with the original C99-FLAG. Arrowheads indicate the position of immunoglobulin G used for co-immunoprecipitation. Data are expressed as means±s.d. of three independent experiments. *P<0.05, **P<0.005, ***P<0.0005 (ANOVA, Scheffe’spost hoctest compared with C99). Full size image Figure 5: Reverse sequence of Aβ1–16 in C99-FLAG exhibited indistinctive cleavage compared with the original C99 substrate. The 1–16 region of C99 was inverted in C99-FLAG substrate (RVC99-FLAG) and we compared its cleavage efficiency with original C99-FLAG ( a ). Underline, inverted sequence of Aβ1–16. C99, RVC99 and Notch substrates were incubated with a γ-secretase fraction at 37 °C for 4 h. ICD-FLAG fragments were separated on a gel, followed by western blotting with anti-FLAG M2 antibody ( b ). C99-FLAG substrate containing a reverse sequence of Aβ1–16 in C99 exhibited indistinctive cleavage compared with original C99-FLAG. Arrow indicates a degradation product of the substrate during purification. Data are expressed as means±s.d. of three independent experiments. *** P <0.0005 (analysis of variance, (ANOVA), Scheffe’s post hoc test compared with C99). NS, not significant. Substrates were immobilized using anti-FLAG M2 magnetic beads and mixed with γ-secretase fractions ( c ). After sufficient washing of co-immunoprecipitates, western blotting was used to visualize and quantify γ-secretase components. RVC99-FLAG showed indistinctive interaction with γ-secretase components compared with the original C99-FLAG. Arrowheads indicate the position of immunoglobulin G used for co-immunoprecipitation. Data are expressed as means±s.d. of three independent experiments. * P <0.05, ** P <0.005, *** P <0.0005 (ANOVA, Scheffe’s post hoc test compared with C99). Full size image Although γ-secretase is widely believed to be a promiscuous protease-cleaving variant of type I membrane proteins, our data clearly demonstrate that γ-secretase possesses substrate preference. This substrate preference was observed even in the γ-secretase fraction from human brain ( Supplementary Figs. S5 and S21 ). This suggests that γ-secretase distinguishes the ectodomain length of substrates by capturing the ectodomain even in the human brain. These findings allowed us to explore the establishment of substrate-specific inhibition of Aβ production. Inhibition of Aβ production by substrate-targeting approach Our data above indicate that γ-secretase captures the ectodomain of the substrate in agreement with the study by Shah et al. [37] , which suggests that blocking interaction of C99 with γ-secretase leads to inhibition of C99 cleavage. To investigate the possibility of substrate-specific inhibition of Aβ production by blocking the ectodomain of C99, we developed C99-blocking agents by employing a DNA library that encodes peptides consisting of 20 randomized amino acids and a cell-free peptide-displaying system ( Supplementary Fig. S6 ) [38] . Cys-rich peptides were panned out by using Aβ1–28 as bait, and we used a CDCYCxxxxCxCxSC motif found in peptides 9–7 and 6–5 as a framework structure with which to improve the inhibitory activity against Aβ production ( Supplementary Fig. S7 ; Fig. 6a ). A subset of 9–7 derivative peptides (#1, #2 and #4) showed striking reduction of Aβ production from the C99-FLAG in the CHAPSO-solubilized γ-secretase assay ( Fig. 6b ; Supplementary Fig. S18 ). We next examined substrate specificity of peptides #1 and #4. As shown in Fig. 6c , these peptides specifically inhibited AICD production from C99-FLAG in a dose-dependent manner. Consistent with substrate specificity of the peptides, dot blot analysis demonstrated that peptide #4 selectively recognized the Aβ1–16 region ( Fig. 6d ; Supplementary Fig. S18 ). BIACORE analysis revealed that peptide #4 with APP633–680 (the flanking region of the beta-cleavage site containing the extracellular domain of C99) had an affinity of ~2.62 μM and that this peptide showed no appreciable binding to Notch1690–1725 (the flanking region of the S2 cleavage site containing the extracelluar domain of V1711 Notch) ( Supplementary Fig. S8 ). 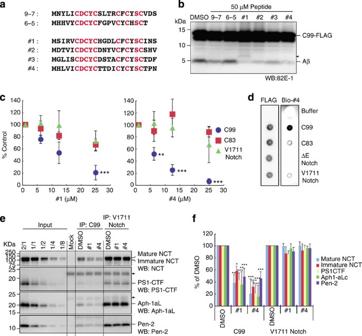Figure 6: Substrate-specific inhibition of γ-secretase-dependent C99 cleavage by C99-binding peptides. Peptide sequence of C99-binding peptides (a). Two peptides (9–7 and 6–5) were panned out using a cell-free peptide-displaying system. The CDCYCxxxxCxCxSC motif (in red) found in peptides 9–7 and 6–5 was used as a skeletal structure to generate 9–7 derivatives (peptides #1 to #4). C99-FLAG substrate was incubated with a CHAPSO-solubilized γ-secretase fraction in the presence of the peptides (b). These peptides inhibited Aβ production. The arrowhead indicates the retardation of Aβ migration caused by peptide #1. Peptides #1 and #4 specifically inhibited AICD production from C99-FLAG in a dose-dependent manner (c). Data are expressed as means±s.d. of three independent experiments. **P<0.005, ***P<0.0005 (analysis of variance (ANOVA), Scheffe’spost hoctest compared with DMSO control). Dot blot analysis of peptide #4 (d). Four picomols of substrates (C99-FLAG, C83-FLAG, V1711 Notch-FLAG and ΔE Notch-FLAG) were placed on nitrocellulose and dehydrated. After blocking with 5% skim milk, the membrane was incubated with biotinylated peptide #4 and streptavidin-conjugated HRP and the peptide bound to the substrates was visualized. Peptide #4 selectively bound to the C99-FLAG. C99-FLAG or V1711 Notch-FLAG was immobilized using anti-FLAG M2 magnetic beads and mixed with a CHAPSO-solubilized γ-secretase fraction in the presence or absence of the peptides (e). Western blotting was used to visualize and quantify γ-secretase components in co-immunoprecipitates. The peptides significantly reduced the interaction of C99 with γ-secretase components compared with the interaction of V1711 Notch. Data are expressed as means±s.d. of three independent experiments (f). *P<0.05, **P<0.005, ***P<0.0005 (ANOVA, Scheffe’spost hoctest compared with DMSO control). Figure 6: Substrate-specific inhibition of γ-secretase-dependent C99 cleavage by C99-binding peptides. Peptide sequence of C99-binding peptides ( a ). Two peptides (9–7 and 6–5) were panned out using a cell-free peptide-displaying system. The CDCYCxxxxCxCxSC motif (in red) found in peptides 9–7 and 6–5 was used as a skeletal structure to generate 9–7 derivatives (peptides #1 to #4). C99-FLAG substrate was incubated with a CHAPSO-solubilized γ-secretase fraction in the presence of the peptides ( b ). These peptides inhibited Aβ production. The arrowhead indicates the retardation of Aβ migration caused by peptide #1. Peptides #1 and #4 specifically inhibited AICD production from C99-FLAG in a dose-dependent manner ( c ). Data are expressed as means±s.d. of three independent experiments. ** P <0.005, *** P <0.0005 (analysis of variance (ANOVA), Scheffe’s post hoc test compared with DMSO control). Dot blot analysis of peptide #4 ( d ). Four picomols of substrates (C99-FLAG, C83-FLAG, V1711 Notch-FLAG and ΔE Notch-FLAG) were placed on nitrocellulose and dehydrated. After blocking with 5% skim milk, the membrane was incubated with biotinylated peptide #4 and streptavidin-conjugated HRP and the peptide bound to the substrates was visualized. Peptide #4 selectively bound to the C99-FLAG. C99-FLAG or V1711 Notch-FLAG was immobilized using anti-FLAG M2 magnetic beads and mixed with a CHAPSO-solubilized γ-secretase fraction in the presence or absence of the peptides ( e ). Western blotting was used to visualize and quantify γ-secretase components in co-immunoprecipitates. The peptides significantly reduced the interaction of C99 with γ-secretase components compared with the interaction of V1711 Notch. Data are expressed as means±s.d. of three independent experiments ( f ). * P <0.05, ** P <0.005, *** P <0.0005 (ANOVA, Scheffe’s post hoc test compared with DMSO control). Full size image To confirm whether peptides #1 and #4 interfere with the interaction between C99 and γ-secretase, we conducted a co-immunoprecipitation assay, performed as shown in Fig. 4c , in the presence of these peptides. C99-binding peptides markedly reduced the interaction of C99 with γ-secretase components compared with the interaction of V1711 Notch ( Fig. 6e,f ; Supplementary Fig. S18 ). Although we could not exclude the possibility that these peptides also reduced the interaction of C99 with free γ-secretase components (that did not participate in the γ-secretase complex), the reduced interaction correlated closely with the inhibition of C99 cleavage. Thus, it is reasonable to interpret that these peptides interfere with the interaction between C99 and γ-secretase complex and suppress the γ- and ε-cleavages of C99, specifically. The ectodomain of C99 is a potential drug target for substrate-specific inhibition of Aβ production. C99-binding peptides suppress β-cleavage of APP Production of C99 is the consequence of β-secretase-dependent cleavage (β-cleavage) of APP (see Fig. 7a ). β-Secretase is also a promising drug target for anti-amyloid therapeutics for reducing C99 production [17] , [18] . However, as in the case of γ-secretase, β-secretase hydrolyses a number of membrane proteins. Thus, substrate-specific inhibition of β-secretase is an ideal approach for anti-Aβ therapeutics. Paganetti et al. [39] demonstrated that the expression of single-stranded intrabodies against the region prior to the β-cleavage site reduced Aβ production. Arbel et al. [40] also reported that antibodies raised against the β-cleavage site (ISEVKMDA) of APP inhibited reduced Aβ production. However, it was unclear whether those antibodies affected β-cleavage directly or indirectly (for example, by alteration of APP trafficking). We established an in vitro β-secretase assay system using an APP-derived fragment (position 633–685 in APP751; referred to as APP633–685-FLAG) and examined the inhibitory effect of peptides #1 and #4 on β-cleavage ( Fig. 7a,b ; Supplementary Fig. S19 ). Peptide #4 attenuated the β-cleavage of the APP633–685-FLAG substrate in a dose-dependent manner ( Fig. 7b,c ). Although we could not detect a statistically significant difference, peptide #1 also tended to reduce the production of Aβ33-FLAG ( Fig. 7b,c ). Interestingly, peptide #1 retarded the mobility of Aβ33-FLAG, as well as of Aβ in the gel, probably due to SDS–stable interaction with Aβ or disturbed gel running ( Fig. 7b,e ; Supplementary Fig. S19 ; see also Fig. 6b and Supplementary Fig. S10b ). We also use a fragment of St6gal 1 (St6gal25–63-FLAG) as another β-secretase substrate to examine substrate-specific inhibition of β-secretase by C99-binding peptides ( Fig. 7d ; Supplementary Fig. S19 ) [24] . None of these peptides inhibited the β-secretase-dependent cleavage of St6gal25–63-FLAG ( Fig. 7e ; Supplementary Fig. S19 ). These data suggest that the inhibitory effect of C99-binding peptides on β-secretase is APP specific. 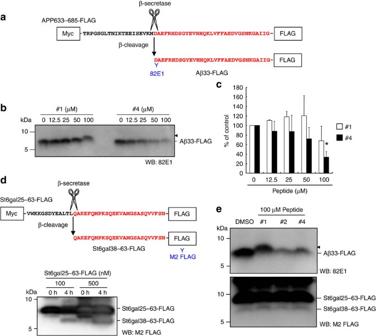Figure 7: C99-binding peptides inhibited β-cleavage of APP in a substrate-specific manner. A fragment of human APP751 (position 633–685) was expressed as a fusion protein with N-terminal Myc and C-terminal FLAG tags inE. coliBL21 and was affinity purified using Anti-FLAG M2 beads. Resultant APP633–685-FLAG was cleaved by β-secretase to produce Aβ33-FLAG (a). Peptide #4 significantly inhibited β-cleavage of the APP633–685-FLAG in a dose-dependent manner (b). The arrowhead indicates the retardation of Aβ33-FLAG migration caused by peptide #1. Data are expressed as means±s.d. of three independent experiments. *P<0.05 (analysis of variance (ANOVA), Scheffe’spost hoctest compared with DMSO control). A fragment of rat St6gal1 (position 25–63, St6gal25–63-FLAG) was incubated with β-secretase to produce St6gal38–63-FLAG (c). C99-binding peptides inhibited β-cleavage of the APP633–685-FLAG (upper panel), but failed to suppress cleavage of St6gal25–63-FLAG (lower panel) (d). The arrowhead indicates the shifted Aβ33-FLAG migration as a probable effect of #1 peptide binding. Figure 7: C99-binding peptides inhibited β-cleavage of APP in a substrate-specific manner. A fragment of human APP751 (position 633–685) was expressed as a fusion protein with N-terminal Myc and C-terminal FLAG tags in E. coli BL21 and was affinity purified using Anti-FLAG M2 beads. Resultant APP633–685-FLAG was cleaved by β-secretase to produce Aβ33-FLAG ( a ). Peptide #4 significantly inhibited β-cleavage of the APP633–685-FLAG in a dose-dependent manner ( b ). The arrowhead indicates the retardation of Aβ33-FLAG migration caused by peptide #1. Data are expressed as means±s.d. of three independent experiments. * P <0.05 (analysis of variance (ANOVA), Scheffe’s post hoc test compared with DMSO control). A fragment of rat St6gal1 (position 25–63, St6gal25–63-FLAG) was incubated with β-secretase to produce St6gal38–63-FLAG ( c ). C99-binding peptides inhibited β-cleavage of the APP633–685-FLAG (upper panel), but failed to suppress cleavage of St6gal25–63-FLAG (lower panel) ( d ). The arrowhead indicates the shifted Aβ33-FLAG migration as a probable effect of #1 peptide binding. Full size image C99-binding peptides inhibited Aβ production in living cells Next, we evaluated the effect of C99-binding peptides on Aβ production in living cells. CHO cells overexpressing APP751, mouse ΔE Notch1 and St6gal1 were cultivated for 48 h in the presence of peptides #1, #2 or #4 (refs 33 , 34 , 41 ). Cell lysates and conditioned media were subjected to western blotting to visualize the levels of Aβ, sAPPβ, C99 and NICD. C99-binding peptides #1 and #4 significantly reduced the levels of Aβ and sAPPβ released from the cells and those of intracellular C99 and Aβ in a dose-dependent manner; however, they showed no alteration of NICD and sAPPα productions ( Fig. 8a ; Supplementary Figs S9 and S22 ). To confirm the substrate-specific inhibition of β-cleavage in this cell model, we evaluated the levels of st6gal1 released by β-secretase-dependent cleavage. Peptides tested in this assay failed to inhibit the release of st6gal1 fragment into the media, indicating that these peptides retained a substrate-specific inhibitory effect on β-secretase even in the cell model ( Supplementary Figs S9 and S22 ). Importantly, reverse sequence peptides failed to inhibit β- and γ-cleavages ( Supplementary Figs S9 and S22 ). We found that biotinylated #4 was markedly incorporated into cells overexpressing APP (7WD10), indicating that striking differences in the visualization of peptide #4 between CHO and 7WD10 reflect the expression of APP ( Fig. 8b ). Our data demonstrate that inhibitory effects of C99-binding peptides on β- and γ-cleavage are essentially dependent on their sequence, rather than on their composition. 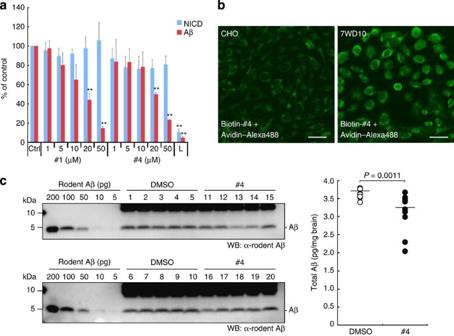Figure 8:In vitroandin vivoefficacy of C99-binding peptides. CHO cells overexpressing APP and mouse Notch1 ΔE were incubated with various amounts of peptides for 48 h (a). Peptides #1 and #4 significantly reduced Aβ production but failed to suppress NICD production in the cells. L, 1 μM L685458. Data are expressed as means±s.d. of three independent experiments. **P<0.005 (analysis of variance (ANOVA), Scheffe’spost hoctest compared with DMSO control). 7WD10, CHO cells overexpressing human APP751 were treated with biotinylated peptide #4 (b). Fixed and permeabilized cells were stained using streptavidin–Alexa488. Robust biotinylated peptide #4 staining was observed in 7WD10, but not in CHO. Bar, 50 μm. Seven-week-old mice were administered peptide #4 (150 mg kg−1d−1) intraperitoneally for 3 days (c). After removal of the brain, endogenous Aβ was extracted from the cortex of one hemisphere, immunoprecipitated using 4G8 antibody and quantified by western blotting. Data are expressed as a scatter plot of data from 10 mice. Bar, median. Significance was assessed using the Mann–WhitneyUtest. Figure 8: In vitro and in vivo efficacy of C99-binding peptides. CHO cells overexpressing APP and mouse Notch1 ΔE were incubated with various amounts of peptides for 48 h ( a ). Peptides #1 and #4 significantly reduced Aβ production but failed to suppress NICD production in the cells. L, 1 μM L685458. Data are expressed as means±s.d. of three independent experiments. ** P <0.005 (analysis of variance (ANOVA), Scheffe’s post hoc test compared with DMSO control). 7WD10, CHO cells overexpressing human APP751 were treated with biotinylated peptide #4 ( b ). Fixed and permeabilized cells were stained using streptavidin–Alexa488. Robust biotinylated peptide #4 staining was observed in 7WD10, but not in CHO. Bar, 50 μm. Seven-week-old mice were administered peptide #4 (150 mg kg −1 d −1 ) intraperitoneally for 3 days ( c ). After removal of the brain, endogenous Aβ was extracted from the cortex of one hemisphere, immunoprecipitated using 4G8 antibody and quantified by western blotting. Data are expressed as a scatter plot of data from 10 mice. Bar, median. Significance was assessed using the Mann–Whitney U test. Full size image C99-binding peptide reduces endogenous cerebral Aβ in mice C99-binding peptide #4, as well as peptides #1 and #2, markedly reduced Aβ production from rodent C99-FLAG substrate in the γ-secretase assay ( Supplementary Figs S10 and S23 ). We also confirmed that these peptides attenuated endogenous production of Aβ in CHO and N2a cells ( Supplementary Figs S11a and S23 ). These results suggest that these peptides are appropriate for testing their efficacy to inhibit Aβ production in animal models expressing rodent APP, although we failed to visualize biotinylated peptide #4 in N2a cells, probably because of the low level of expression of endogenous APP in the cells and insufficient affinity of the peptide for APP, compared with anti-Aβ antibodies ( Supplementary Fig. S11b ; see also Supplementary Fig. S8 ). Wild-type mice are ideal models with which to examine the efficacy of APP-targeting drugs because of their moderate endogenous expression of APP, compared with human APP transgenic mice. To assess their inhibitory efficiency in vivo , peptide #4 was administered to wild-type mice (150 mg kg −1 d −1 intraperitoneal) for 3 days. Animals were killed and their brain extracts were analysed by immunoprecipitation with 4G8 and western blotting with anti-rodent Aβ antibody. We found that levels of endogenous cerebral Aβ in the mice administered with peptide #4 were significantly reduced ( Fig. 8c ; Supplementary Fig. S20 ). To investigate whether C99-binding peptide penetrates through the brain, we intraperitoneally administered fluorescein isothiocyanate-labelled peptide #4 into mice and examined the brain distribution of the peptide. Although the peptide was not detected in individual neurons, as in the case of N2a cells shown in Supplementary Fig. S11b , we observed faint fluorescence of the peptide in the cortex and hippocampus (CA1 and DG) and its robust signal in the choroid plexus of the lateral ventricle of brains administered the peptide ( Supplementary Fig. S12 ). Preclinical studies of passive Aβ immunotherapy have proposed phagocytosis of antibody-opsonized Aβ by microglia as a potential mechanism for Aβ clearance in the brain [42] . It seems reasonable to suppose that a certain amount of the peptide enters the brain in our current study, as in the case of anti-Aβ antibodies in passive Aβ immunotherapy. Substrate-specific inhibition of γ-secretase remains an unsolved important issue for overcoming AD. Uncovering the mechanism of substrate preference and substrate recognition of γ-secretase is a key step to establishing substrate-specific inhibition of Aβ production. The requirement for γ-secretase cleavage was first reported by Struhl and Adachi [43] . They applied a reporter gene assay with various transmembrane proteins containing different ectodomain lengths in an insect model and found that γ-secretase cleavage was independent of particular sequences in transmembrane domains. They also demonstrated that transmembrane proteins containing ectodomains smaller than 50 residues were efficiently cleaved, compared with those containing over 50-residue extracellular domain, by this protease. Here, we also show that γ-secretase preferentially cleaves substrates containing a short ectodomain and the cleavage is not susceptible to the total substrate length or C-terminal length of the substrate. Their pioneering study and our current study take a similar view. However, a large discrepancy exists between the two studies. The previous study reported that transmembrane proteins with fewer than 50 extracellular amino acids were cleaved with similar efficiency to that of S2 cleaved Notch containing 15 extracellular amino acids [43] . According to the pioneering study, cleavage efficiency of the substrates used in our study is supposed to be similar, because the number of extracellular amino acids of our substrates is in the range of 12–28 ( Figs 1 and 2 ). By contrast, our straightforward cleavage analyses showed that γ-secretase preferentially cleaved substrates containing a short ectodomain in three different transmembrane proteins (APP, APLP2 and Notch) ( Fig. 2 ). Our ectodomain-swapping experiments also indicated that γ-secretase distinguishes the ectodomain length, even in substrates containing fewer than 30 extracellular amino acids ( Fig. 4b,c ; Supplementary Figs S4 and S5 ). The reporter gene assay is a powerful and reliable tool for detecting the presence of molecules liberated to activate downstream gene expression. However, it is noteworthy that this assay is indirect, not accurately quantitative and easily becomes saturated. It is likely that the indirect approach in the pioneering study was insufficiently sensitive to detect the difference of cleavage efficiency between substrates containing an ectodomain smaller than 50 residues. In addition, direct substrates containing over 50 extracellular amino acids have not been reported in cultured cells and physiological conditions, except for experimentally generated substrates [43] , [44] . It is likely that transmembrane proteins with such long ectodomains can be substrates after N-terminal truncation in vivo . At present, the known ectodomain size of direct γ-secretase substrates is in range of 12–35 residues [12] , [19] , [45] , [46] , [47] . It is very important to use direct substrates containing a native ectodomain for investigation of the substrate preference of γ-secretase. Our data indicated that short ectodomain substrates (C83 and V1711 Notch) increased interaction with γ-secretase components in co-immunoprecipitation experiments ( Fig. 4c ; Supplementary Figs S4 and S5 ). Although we could not exclude the possibility that unassembled γ-secretase components solely prefer to interact with short ectodomain substrates, cleavage efficiency of the substrates correlated with the interaction. Thus, it is an entirely reasonable interpretation that the γ-secretase complex preferentially interacts with the short ectodomain substrates. However, we observed that the levels of immature nicastrin co-immunoprecipitated with C99 and V1711 Notch substrates were similar to each other. It was reported that recombinant nicastrin expressed in insect cells solely bound to C99 and that co-immunoprecipitant with C99 from MEF contained immature nicastrin and its mature form [37] . This suggests that unassembled immature nicastrin is able to interact with substrates. On the other hand, Herreman et al. [48] demonstrated that γ-secretase activity was not influenced by the glycosylation status of nicastrin. Their report suggests that the γ-secretase complex containing immature nicastrin can recognize and cleave substrates. According to the report by Herreman et al. [48] , it is possible to assume that a γ-secretase complex containing immature nicastrin lacks in substrate preference and that the glycosylation status of nicastrin in the complex may be crucial for the substrate preference of γ-secretase. In this study, we demonstrated that γ-secretase favours short ectodomain substrates. However, it is still unclear how and why this enzyme preferentially recognizes substrates containing a short ectodomain. In good agreement with the finding by Shah et al. [37] , our data support the idea that γ-secretase captures the N terminus of the substrate. It may safely be assumed that the N terminus of a substrate containing a long ectodomain is too distant from γ-secretase to be captured by this enzyme ( Fig. 9a ) [49] . Recently, Watanabe et al. [50] reported that transmembrane domains 2 and 6 of presenilin 1 have a role in the formation of an initial substrate-binding site of γ-secretase. It is reasonable to consider that the extracellular interaction of γ-secretase with its substrates is critical for substrate preference of this enzyme, rather than the initial substrate binding in the transmembrane region of γ-secretase. 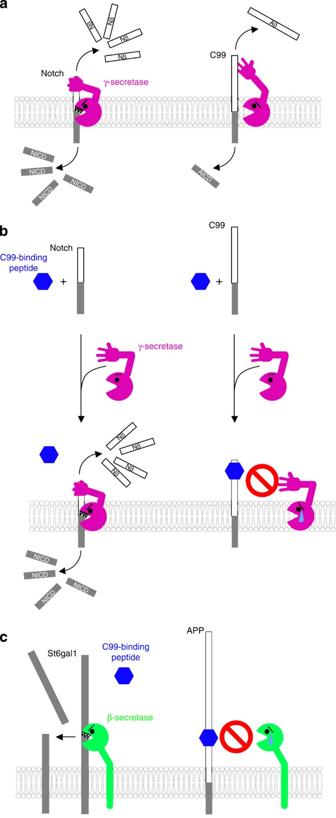Figure 9: Models for substrate preference of γ-secretase and inhibition of APP cleavage by C99-binding peptide. γ-Secretase easily captures the N terminus of substrates containing a short ectodomain, such as C83, R678 APLP2 and V1711 Notch, which results in increased cleavage efficiency of the substrates (a, left). By contrast, the N terminus of substrates containing a long ectodomain (C99, M664 APLP2 and ΔE Notch) is located distantly to γ-secretase, leading to decreased interaction between the substrate and γ-secretase and inefficient cleavage (a, right). The C99-binding peptide interferes with interaction of γ-secretase with C99, but not Notch (b). The C99-binding peptide binds to the flanking region of the APP β-cleavage site and inhibits APP processing by β-secretase (c). C99-binding peptide fails to interfere with interaction of β-secretase with St6gal1. Figure 9: Models for substrate preference of γ-secretase and inhibition of APP cleavage by C99-binding peptide. γ-Secretase easily captures the N terminus of substrates containing a short ectodomain, such as C83, R678 APLP2 and V1711 Notch, which results in increased cleavage efficiency of the substrates ( a , left). By contrast, the N terminus of substrates containing a long ectodomain (C99, M664 APLP2 and ΔE Notch) is located distantly to γ-secretase, leading to decreased interaction between the substrate and γ-secretase and inefficient cleavage ( a , right). The C99-binding peptide interferes with interaction of γ-secretase with C99, but not Notch ( b ). The C99-binding peptide binds to the flanking region of the APP β-cleavage site and inhibits APP processing by β-secretase ( c ). C99-binding peptide fails to interfere with interaction of β-secretase with St6gal1. Full size image Based on the mechanism of substrate recognition by γ-secretase, we generated C99-binding peptides to interfere with the interaction of C99 with γ-secretase. Our results are consistent with the previous report that chemical or antibody-mediated blocking of the C99 N terminus reduced interaction with free nicastrin and production of AICD [37] . Our data demonstrate that blocking the ectodomain of C99 by its binding peptides inhibits not only the interaction with nicastrin but also that with γ-secretase. The most prominent feature of our substrate-targeting approach is that C99-binding peptides exhibited substrate-specific inhibition of β-cleavage of APP as well as γ-cleavage of C99 even in a cell-based assay ( Fig. 9b,c ). We believe this strategy, which kills two birds with one stone, is a potent approach for substrate-specific dual inhibition of β- and γ-secretases. Interestingly, we found that WO2, an antibody raised against the N terminus of Aβ, was able to inhibit Aβ production, as do antibodies 82E1 and 6E10 ( Supplementary Figs S13 and S23 ). Recently, the structure of the WO2–Aβ complex was determined by Miles et al. [51] Based on this inhibition, generating small compounds that specifically bind to the N terminus of C99 (or Aβ) represents a valid approach for developing a disease-modifying strategy to combat AD. Cell culture CHO, HEK293 and N2a cells were obtained from ATCC and cultured in Dulbecco’s modified Eagle’s medium (Sigma) supplemented with 10% fetal bovine serum (Invitrogen) and penicillin/streptomycin (Invitrogen) [51] . For stable transfectant, 7WD10, G418 (Wako) was added to the culture medium at a concentration of 200 μg ml −1 (ref. 52 ). Antibodies The antibodies used for protein detection in this study were as follows: anti-human Aβ antibodies 82E1 (1/100 dilution in TBS containing 0.1% Tween; IBL); 6E10 (1/1,000 in TBS containing 0.1% Tween; Covance); 4G8 (1/1,000 in TBS containing 0.1% Tween; Covance); anti-rodent Aβ antibody 28055 (1/100 in TBS containing 0.1% Tween; IBL); anti-sAPPβ antibody 18957 (1/100 in TBS containing 0.1% Tween; IBL); anti-NICD antibody #2421 (1/100 in TOYOBO Can Get Signal; Cell Signalling Technology); anti-St6gal1 antibody 18983 (1/100 in TBS containing 0.1% Tween; IBL); anti-nicastrin antibody N1660 (1/1,000 in TBS containing 0.1% Tween; Sigma); anti-Aph-1a loop antibody O2F1 (1/1,000 in TOYOBO Can Get Signal; Covance); anti-PS1–CTF anti-serum, anti-PS1–NTF anti-serum (1/3,000 in TBS containing 0.1% Tween; gifts from Drs T. Iwatsubo and T. Tomita, The University of Tokyo); anti-Pen-2 antibody (1/3,000 in TBS containing 0.1% Tween; a gift from Dr A. Takashima, National Center for Geriatrics and Gerontology); anti-AICD anti-serum UT-18 (1/5,000 in TBS containing 0.1% Tween; a gift from Dr T. Suzuki, Hokkaido University); and anti-FLAG M2 antibody (1/1,000 in TBS containing 0.1% Tween; Sigma). For high-sensitivity detection on western blotting, nitrocellulose membrane Protran BA83 (GE Healthcare) was soaked in phosphate-buffered saline after transferring protein and boiled for 5 min in an aluminium boiling apparatus (Can Do, Tokyo). WO2 (Millipore) was used at a concentration of 200 nM for suppression of Aβ production (see Supplementary Fig. S13 ). γ-Secretase substrates γ-Secretase substrates were expressed as fusion proteins with an APP signal peptide and the Profinity eXact tag (Bio-Rad) in sf9 cells by using Bac-to-Bac Baculovirus Expression System (Invitrogen) ( Fig. 1 ). Sf9 cells were infected with recombinant baculovirus according to the manufacturer’s instructions. Infected cells were harvested after 36 h and resuspended in 50 mM PIPES (pH 7.0), 250 mM sucrose. The cell suspension was mixed with an equal amount of lysis buffer (50 mM PIPES (pH 7.0), 250 mM sucrose, 2% NP40 and 2 × protease inhibitor cocktail (Roche Diagnostics)) and incubated on ice for 1 h. After ultracentrifugation at 100,000 × g centrifugation for 1 h, the supernatant was agitated overnight with Profinity eXact (S189 subtilisin-immobilized) resin (Bio-Rad). The Profinity eXact tag protein purification system offers purification of recombinant proteins with a native N terminus. Once Profinity eXact-tagged γ-secretase substrates were captured using S189 subtilisin-immobilized resin, addition of sodium fluoride triggered precise cleavage at the C terminus of the cleavage-recognition sequence and the release of substrates with a bona fide N terminus. Substrate purification was performed according to the manufacturer’s instructions. Purified substrates were recaptured using anti-FLAG M2 agarose beads (Sigma) for concentration and eluted by addition of 0.2 M glycine (pH 2.7) and 0.3% NP40. A one-tenth volume of 3 M Tris-HCl (pH 8.0) was added to the eluted substrates for neutralization and quantified [35] . Five-residue N-terminal sequence of each substrate was confirmed by Edman degradation. γ-Secretase assay The microsomal fraction of CHO cells was solubilized by adding an equal volume of 2 × NK buffer (50 mM PIPES (pH 7.2), 250 mM sucrose, 1 mM EGTA, 2% CHAPSO, 1 mM DIFP, 20 μg ml −1 antipain, 20 μg ml −1 leupeptin, 10 μg ml −1 TLCK, 10 mM phenanthroline and 2 mM thiorphan). The supernatant obtained after 100,000 × g centrifugation for 1 h was used as a source of γ-secretase. The CHAPSO lysate was diluted with three volumes of the dilution buffer (50 mM PIPES (pH 7.2), 250 mM sucrose, 1 mM EGTA, 1 mM DIFP, 10 μg ml −1 antipain, 10 μg ml −1 leupeptin, 10 μg ml −1 TLCK, 5 mM phenanthroline and 1 mM thiorphan). A 1/10th volume of 1% phosphatidylcholine (solubilized in 1% CHAPSO) was added to the diluted γ-secretase reaction. γ-Secretase substrates were incubated with the diluted CHAPSO lysate at 37 °C for 4 h in the presence or absence of the peptides or antibodies. Western blotting was used to analyse the production of Aβ, ICD and components in the incubated reaction mixtures (see also Antibodies above) [32] . Human cortical specimens for γ-secretase assay were obtained from brains that were removed, processed and stored at −80 °C within 12 h postmortem at the Brain Bank at Tokyo Metropolitan Institute of Gerontology. For all brains registered at the bank, we obtained written informed consent for their use for medical research from patients or their family members. The human brains were subjected to solubilization in CHAPSO as described above. This study was approved by the ethic committee at Tokyo Metropolitan Institute and Doshisha University. Co-immunoprecipitation of γ-secretase substrates γ-Secretase substrate was immobilized on anti-FLAG M2 magnetic beads by incubating them together at 4 °C for 2 h. The beads were mixed with the diluted CHAPSO lysate at 4 °C overnight in the presence or absence of the peptides. After sufficient washing of co-immunoprecipitates, western blotting was used to visualize γ-secretase components. Selection of binding peptides A DNA library was constructed from synthetic oligonucleotides, which included ATG(NNT) 20 or ATG(NNK) 20 (N is A, C, G or T, and K is G or T) as a randomized peptide-encoding region. The NNT-type was added in the same amount as the NNK-type to increase the proportion of Cys and Tyr and to decrease the appearance of stop codons. The DNA library (100 pmol) was used for transcription and the resultant mRNA library was employed as a template for a covalently linked peptide or protein-displaying system [38] . Peptide-displaying molecules were incubated with 2.6 μM of Aβ1–28 immobilized at its biotinylated C terminus on Dynabeads M-280 Streptavidin (Invitrogen) for 1 h at ambient temperature. After washing the beads, the binding molecules were recovered by heating at 95 °C and subjected to PCR for preparation of templates for the next round. The concentration of binding molecules was repeated six times in this manner and was followed by three rounds with the fourfold-diluted bait. Recovery of templates increased with increasing number of selection rounds, and five clones after the 6 th round and seven clones after the 9 th round were sequenced. Two sequences sharing a CDCYCxxxxCxCxCxSC motif were semi-randomized by the secondary DNA library including ATG(NNT) 4 TGTGATTGTTATTGT(NNT) 4 TGTTHTTGTBATTHTTGT(NNT) 3 , where H is A/C/T and B is C/G/T. Selection from the secondary library was performed in the same way as done in the 7 th round in the initial selection except that the incubation temperature was 37 °C. After five rounds of selection and cloning, four derivative peptides were identified ( Fig. 6a ). Dot blot analysis Solutions containing γ-secretase substrate (4 pmol) were placed on a nitrocellulose membrane and dehydrated. After blocking with 5% skimmed milk for 30 min, the membrane was incubated with biotinylated peptide #4 for 2 h at room temperature. The membrane was incubated with streptavidin-conjugated HRP, and the peptide bound to substrate was visualized using an ECL system. Biacore analysis Affinity of #4 peptide was determined by kinetic analysis of Biacore T100 (GE healthcare). APP633–680-His tag (5 μM in phosphate-buffered saline) was immobilized to a NTA sensor tip according to the manufacturer’s instructions. A continuous flow of HBS N buffer containing 2% DMSO (10 mM HEPES (pH7.4), 150 mM NaCl, 2% DMSO) was maintained over the sensor surface at 20 μl min −1 . Kinetic experiments of #4 peptide were performed at 25 °C. S #4 peptide was serially diluted in the buffer to working concentrations. The peptide was injected for 6 min and dissociation was monitored for 4 min. β-Secretase assay A fragment of human APP (position 633–685 in APP751) was expressed as a fusion protein with N-terminal Myc and C-terminal FLAG tags in Escherichia coli BL21 and was affinity-purified using ANTI-FLAG M2 beads. The purified fragment (referred to as APP633–685-FLAG) was quantified by CBB staining after gel electrophoresis. APP633–685-FLAG (50 nM) was incubated with β-secretase (Sigma) for 4 h according to the manufacturer’s instructions, in the presence or absence of the peptides. β-cleaved C-terminal fragments (Aβ33-FLAG) from APP633–685-FLAG were visualized and quantified using the 82E1 antibody (IBL). Inhibition of Aβ production in the cell-based assay 7WD10, CHO cells overexpressing APP751, mouse Notch1 ΔE and St6gal1 were inoculated at a density of 1.5 × 10 5 cells per well in a 24-well plate. Subsequently (20–24 h later) [24] , [33] , [34] , [41] , the culture medium was replaced with medium containing various concentrations of peptides. After 48 h incubation, the conditioned medium and cells were collected and the Aβ, sAPPβ, C99, NICD and St6gal1 released were quantified by western blotting. After the cells were cultivated in medium containing biotinylated peptide #4 for 48 h and fixed in 10% formaldehyde, they were permeabilized by 1% Triton X-100 treatment and incubated with Alexa488-conjugated streptavidin; confocal scanning laser microscopy was used to visualize peptides in the cells. Inhibition of rodent Aβ production in CHO and N2a cells N2a Cells were obtained from ATCC and inoculated at a density of 1.5 × 10 5 cells per well in a 24-well plate. Subsequently (20–24 h later), the culture medium was replaced with a chemically defined, animal-component-free medium, CD-AF (Sigma), in the presence or absence of peptides. After 48 h incubation, conditioned medium was collected, and immunoprecipitation with 4G8 followed by western blotting with anti-rodent Aβ antibody 28055 (IBL) was used to quantify the rodent Aβ. Intraperitoneal administration of the peptide Animal experiments were approved by the Doshisha University animal experimental committee review. Peptide #4 (50 μl of 20 mM) was administered to wild-type mice (C57BL/6 N Cr Slc, female, 7 weeks) intraperitoneally for 3 days (equivalent to 150 mg kg d −1 ). In parallel, vehicle-treated control mice were administered DMSO intraperitoneally. After removal of the brain, the cortex from one hemisphere was homogenized, extracted with a 20 × volume of TBS containing 1% NP-40 and centrifuged at 100,000 × g for 1 h. The supernatant (1 ml) was subjected to immunoprecipitation with 4G8 and to western blotting with anti-rodent Aβ antibody 28055 (IBL) to quantify the rodent Aβ. Data were analysed using Mann–Whitney non-parametric statistics to assess significance. Fluorescein isothiocyanate-labelled peptide #4 was administered to the wild-type mice for 3 days. After perfusion fixation, brains were fixed in 10% formaldehyde for 2 days and 100 μm-thick coronal sections processed by brain slicer (Linearslicer Pro7) were examined by confocal scanning laser microscopy to visualize the peptide. How to cite this article: Funamoto, S. et al. Substrate ectodomain is critical for substrate preference and inhibition of γ-secretase. Nat. Commun. 4:2529 doi: 10.1038/ncomms3529 (2013).